Direct optical sensing of single unlabelled proteins and super-resolution imaging of their binding sites Detection of single analyte molecules without the use of any label would improve the sensitivity of current biosensors by orders of magnitude to the ultimate graininess of biological matter. Over two decades, scientists have succeeded in pushing the limits of optical detection to single molecules using fluorescence. However, restrictions in photophysics and labelling protocols make this technique less attractive for biosensing. Recently, mechanisms based on vibrational spectroscopy, photothermal detection, plasmonics and microcavities have been explored for fluorescence-free detection of single biomolecules. Here, we show that interferometric detection of scattering (iSCAT) can achieve this goal in a direct and label-free fashion. In particular, we demonstrate detection of cancer marker proteins in buffer solution and in the presence of other abundant proteins. Furthermore, we present super-resolution imaging of protein binding with nanometer localization precision. The ease of iSCAT instrumentation promises a breakthrough for label-free studies of interactions involving proteins and other small biomolecules. There are more than 2,000 proteins secreted by the human body at concentrations that are below the detection limit of the current commercial biosensors [1] . To achieve a sufficient sensitivity for early and robust diagnosis of health hazards such as cancer and lethal infectious diseases, scientists have explored a fury of strategies based on mechanical [2] , electrochemical [3] and optical [4] , [5] interactions. The ultimate performance would be to count the analyte molecules one at a time. Furthermore, a practical biosensor would ideally detect the molecule of interest directly and without the need for labelling, amplification or sophisticated architectures. A well-established approach for label-free detection is via the vibrational signatures of molecules, for example via Raman spectroscopy. This method has an exquisite selectivity, but single-molecule sensitivity has only been reached by enhancing the Raman cross-section in the near field of surfaces [6] or tips [7] . A common alternative strategy relies on the detection of the refractive index change due to analyte binding. The oldest and commercially available implementation of this technique records the shift of the plasmon resonance of a gold-coated prism [8] , whereby the specificity and selectivity are provided by surface chemistry [9] . While submonolayer detection is readily achievable in such a device, a single molecule does not manifest a significant change in the refractive index of the sensor medium. To increase the sensitivity, confined modes of plasmonic nanostructures [10] , [11] , [12] and dielectric microresonators [13] , [14] have been investigated, but these techniques are intrinsically limited. First, there is a compromise between the size of the sensor active area and its sensitivity. Higher sensitivity comes through confined intensity distributions and, thus, at the cost of more restricted active area, fewer binding receptors and thinner functionalization [15] . Second, the strong confinement in hotspots is accompanied by a large gradient of sensor response over its active area. As a result, a clear ‘yes–no’ detection is not possible. Furthermore, no spatial information is available about the location of the individual proteins. These shortcomings make it very difficult to characterize the performance of a sensor in a quantitative and robust fashion [16] , [17] . Indeed, the recent reports of single-protein sensitivity have relied on consistency arguments and comparisons with theoretical simulations [11] , [12] , [14] . In this work we report on the direct label-free detection and imaging of individual proteins via the interference of the light created by Rayleigh scattering and the reflection of the incident laser beam [18] , [19] , [20] . Previously, we have used this method (interferometric detection of scattering (iSCAT)) to visualize unlabelled viruses [21] . However, the extension of iSCAT to the detection of single proteins is a nontrivial task because the expected signal, which is about thousand times smaller than that of a virus, is much smaller than the intensity fluctuations originating from the illumination and other scattering sources. In what follows, we show that it is possible to overcome these challenges and detect single proteins of size <60 kDa in a simple and direct arrangement in pure buffer as well as in a mixed sample. 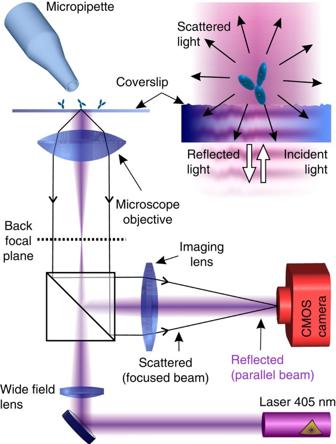Figure 1: Experimental configuration of the interferometric scattering biosensor. Laser light is focused on the back focal plane of a microscope objective. The focal plane of the imaging lens coincides with the back focal plane of the objective. A pulled capillary is used as a micropipette to deliver the analyte locally to the field of view of the microscope. The inset illustrates a zoom of the interactions of the incident, reflected and scattered light waves. Principles of iSCAT detection and sensitivity Figure 1 displays our experimental setup. A laser beam illuminates a glass substrate, and its partial reflection at the substrate–water interface is used as the reference for a homodyne interferometric detection [18] , [20] . Molecules adsorbed on the substrate and any optical surface inhomogeneities generate scattering, which is collected by the microscope objective (see the inset in Fig. 1 ). The reference and scattered components reach a CMOS camera as planar and converging spherical waves, respectively. Because the two optical fields are coherent, they interfere. It is, however, worth mentioning that the common-path nature of this interferometer makes it extremely stable. The detected power ( P det ) is given by Figure 1: Experimental configuration of the interferometric scattering biosensor. Laser light is focused on the back focal plane of a microscope objective. The focal plane of the imaging lens coincides with the back focal plane of the objective. A pulled capillary is used as a micropipette to deliver the analyte locally to the field of view of the microscope. The inset illustrates a zoom of the interactions of the incident, reflected and scattered light waves. Full size image Here, P inc is the incident power, r is the field reflectivity of the glass–water interface, ϕ denotes a phase (mainly determined by the Gouy phase shift [18] ), and the unitless parameter s is related to the particle scattering cross-section and thus polarizability. While the second term ( P scat ) describes the scattering power of the object, the third term ( P int ) represents the beating of the reference (local oscillator) and scattered fields. In the past, the general wisdom has been that the light scattered by a single protein far from any optical resonances would be too small to detect. Thus, before we present our results we scrutinize the orders of magnitude involved. The strength of Rayleigh scattering by a subwavelength nano-object is determined by the incident electric field and its polarizability ( α ), or, equivalently, cross-section ( σ ). Textbook formulae and provide estimates of these quantities, where V is the object volume, n s its refractive index, n m the refractive index of the surrounding medium and λ the illumination wavelength. For a small biomolecule such as albumin with a molecular weight of 65 kDa, effective scattering radius of 3.7 nm (ref. 22 ) and refractive index of 1.44, one obtains σ =10 11 μm 2 at λ =405 nm in an aqueous environment. It follows that an incident power of P inc (in units of photons per second) yields ( σ / A ) P inc scattered photons per second, where we take the characteristic area A associated with the detection of a single protein to be the area of a diffraction-limited spot (DLS). Assuming ideal collection efficiency, no detection losses and A = π (100 nm) 2 , the power registered on the detector is P scat =(3 × 10 −10 ) P inc . This is to be compared with the power of the reference beam P ref =(6 × 10 −3 ) P inc for r 2 =6 × 10 −3 at the water–glass interface. The divide of >10 7 between P scat and P ref puts a severe limitation on the dynamic range of a real detector and renders their simultaneous measurement very difficult. However, the third term in equation (1) corresponding to remains as large as P int =(3 × 10 −6 ) P inc =(5 × 10 −4 ) P ref . Hence, we express the iSCAT signal originating from a nano-object in terms of the contrast . The visibility of P int over P ref depends on the noise level of the latter. In the optimal situation, where the intensity fluctuations are dictated by the photon shot noise, the condition for deciphering P int within integration time τ becomes . Therefore, detection of a small protein in τ =100 ms should be possible for P inc >10 10 photons s −1 DLS −1 , corresponding to 5 nW focused to a DLS. The absolute contrast of iSCAT and, thus, the total number of photons on the detector can be adjusted through the reflectivity r (ref. 18 ). However, if the measurement is shot-noise limited, the dependence of the visibility of the iSCAT signal on r drops out because both the shot noise and the interference term are linearly proportional to r . In a realistic laboratory experiment, losses in the collection of scattered light through the optical elements and in the detector call for a larger power. The actual parameters and considerations of our experiment can be found in the Methods section. Here, it suffices to note that we performed our measurements at the rate of 3,000 frames per second under P inc =15 μW per DLS. We also emphasize that the corresponding intensity is many orders of magnitude away from the damage threshold of biological matter. 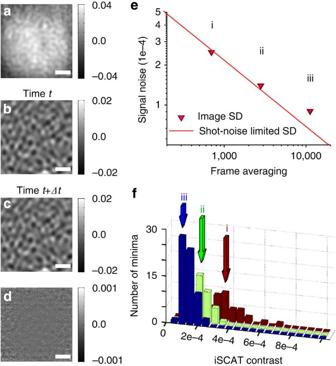Figure 2: Principle of background subtraction. (a) Raw image fluctuations as measured on the camera. (b,c) Two images of surface roughness recorded with a temporal offset of Δt=300 ms after correction for the illumination wavefront. (d) The shot-noise-limited image resulting from the subtraction of (b) and (c). Scale bar, 1 μm. (e) The triangles show the standard deviation of image noise measured for running averages of 700 (i), 2,800 (ii) and 11,200 (iii) frames, The solid line plots a theoretical limit of the shot noise considering the experimentally recorded intensity noise of the CMOS camera. (f) Histograms of noise local minima (iSCAT contrast) detected in the images analysed in (e). Accounting for the background Figure 2a shows a typical iSCAT camera image of a naked substrate. The observed large contrast fluctuations of up to 8% hamper the identification of a single protein. One source of the observed intensity variations is the wavefront inhomogeneity of the incident laser beam. To avoid this issue, previously we used laser beam scanning [18] , [21] . An important feature of the new set-up described in Fig. 1 is that it operates in the wide-field mode, which allows for fast, efficient and parallel sensing over a large area. To eliminate the effect of wavefront corrugations in this imaging mode, we modulated the lateral position of the sample by a few hundred nanomaters using a piezoelectric scanner and used a lock-in principle to extract the optical response of the sample. Figure 2: Principle of background subtraction. ( a ) Raw image fluctuations as measured on the camera. ( b , c ) Two images of surface roughness recorded with a temporal offset of Δ t =300 ms after correction for the illumination wavefront. ( d ) The shot-noise-limited image resulting from the subtraction of ( b ) and ( c ). Scale bar, 1 μm. ( e ) The triangles show the standard deviation of image noise measured for running averages of 700 (i), 2,800 (ii) and 11,200 (iii) frames, The solid line plots a theoretical limit of the shot noise considering the experimentally recorded intensity noise of the CMOS camera. ( f ) Histograms of noise local minima (iSCAT contrast) detected in the images analysed in ( e ). Full size image The resulting image is shown in Fig. 2b and reveals that surface corrugations of the glass coverslip and possibly small local variations in the refractive index fluctuations amount to an iSCAT contrast of the order of 4 × 10 −2 , which is still much larger than the expected contrast of a single protein. In earlier experiments on the absorption of single-dye molecules, we eliminated these fluctuations by index matching a polymer film with immersion oil [20] , but this solution is not viable in a biosensing arrangement. Here, we take advantage of the fact that the introduction of analyte particles in a typical biosensor is an inherently dynamic process, so that each particle is encoded by its arrival time. As a result, subtracting consecutive images can reveal new particles. This strategy has also been used in imaging the diffusion of nanoparticles such as viruses [21] . However, single-protein detection is a much more challenging task because the iSCAT contrast of a protein can be compromised by any residual signal modulation or fluctuation. To demonstrate that we can eliminate all systematic signal fluctuations, we now examine two iSCAT images of a glass surface roughness recorded at a time interval Δ t as shown in Fig. 2b,c . The resulting difference image displayed in Fig. 2d is, indeed, very flat. To investigate the noise limit in this differential image, in Fig. 2e we plot the standard deviation (SD) of the image for averaging 700 (i), 2,800 (ii) and 11,200 (iii) frames. We find that our detection is very close to the theoretical shot-noise limit depicted by the solid line, although at very long integration times mechanical drifts and instabilities of the set-up lead to imperfect background subtraction and give rise to fluctuations that dominate the shot noise. To provide more insight into the behaviour of signal variations, in Fig. 2f we also present histograms of the local minima from a series of 300 different images averaged over 700, 2,800 and 11,200 frames. It is clear that longer integration times reduce the noise, allowing for a detection limit of ~2 × 10 −4 . We emphasize that accounting for background is often the biggest challenge in achieving ultrasensitive detection. In fact, the key steps in pushing the limit of fluorescence microscopy from the detection of small beads in the 1980s [23] to the single-molecule level in the early 1990s [24] also concerned mastering the background fluorescence originating from samples and optical elements. 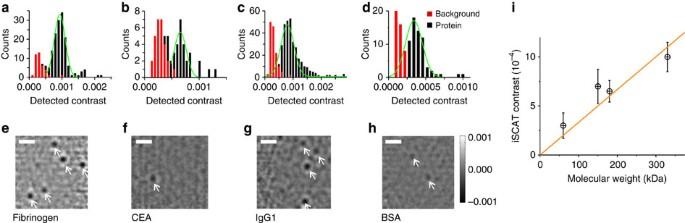Figure 3: iSCAT images and histograms for four different proteins. A histogram of the contrasts measured prior to (background, red) and during (black) detection. (a) Fibrinogen; (b) CEA; (c) IgG1; (d) BSA. Examples of differential images are shown in (e) for fibrinogen, (f) for CEA, (g) for IgG1 and in (h) for BSA. Individual molecules are marked with arrows. Scale bar, 1 μm. (i) Plot of the iSCAT contrast (histogram peak) as a function of the molecular weights of 65, 150, 180 and 340 kDa for BSA, IgG1, CEA and fibrinogen, respectively. Error bars indicate the FWHM of corresponding histograms. Detection of single proteins Figure 3e–h presents examples of differential images after solutions of fibrinogen, carcinoembryonic antigen (CEA), mouse immunoglobulin (IgG1) and bovine serum albumin (BSA) were introduced to the vicinity of a surface activated by N -hydroxysuccinimide (NHS). The images were created using averages of 700 frames for fibrinogen, IgG1 and CEA, and 11,200 frames for BSA. Several well-defined diffraction-limited iSCAT spots in Fig. 3e–h reveal typical contrasts ranging from 3 × 10 −4 for BSA to 1 × 10 −3 for fibrinogen, which is well above the detection limit characterized in Fig. 2f . Figure 3: iSCAT images and histograms for four different proteins. A histogram of the contrasts measured prior to (background, red) and during (black) detection. ( a ) Fibrinogen; ( b ) CEA; ( c ) IgG1; ( d ) BSA. Examples of differential images are shown in ( e ) for fibrinogen, ( f ) for CEA, ( g ) for IgG1 and in ( h ) for BSA. Individual molecules are marked with arrows. Scale bar, 1 μm. ( i ) Plot of the iSCAT contrast (histogram peak) as a function of the molecular weights of 65, 150, 180 and 340 kDa for BSA, IgG1, CEA and fibrinogen, respectively. Error bars indicate the FWHM of corresponding histograms. Full size image Since the iSCAT signal of all individual proteins of a certain type should be the same within our flat field of view, we expect a narrow distribution of the observed contrasts as long as the arrival rate of the analyte is lower than the acquisition rate. To examine our data in this respect, we searched the recorded differential images for local minima that appeared over an area of one point-spread function. Fig. 3a–d displays the histograms of the magnitudes of the iSCAT minima obtained prior to (red) and during (black) the injection of the analyte. In each histogram, a clear peak (black) distinguishes the signal from the background (red) contribution. The fact that the width of the signal distribution is always much smaller than its peak value and that each distribution rapidly falls at larger contrasts lets us attribute each peak to the contrast of a single protein. The small number of occurrences at the large tails of the distributions indicates rare events of clusters of two or more proteins. Full-length videos of the iSCAT detection of fibrinogen, immunoglobulin IgG1 and BSA are shown in Supplementary Movies 1, 2, and 3 , respectively. In Fig. 4a we present a few typical frames of the first video. Furthermore, in Fig. 4b–d we illustrate the temporal kinetics of fibrinogen, IgG1 and BSA detection presented in Supplementary Movies 1, 2, and 3 , respectively. In each case, the kinetics starts with a stable baseline with none or only few molecular bindings. After the sample is flowed towards the sensor surface, a stable binding rate is established until the flow is stopped and the kinetics levels off. Minor irregularities are most probably due to small fluctuations of the flow. 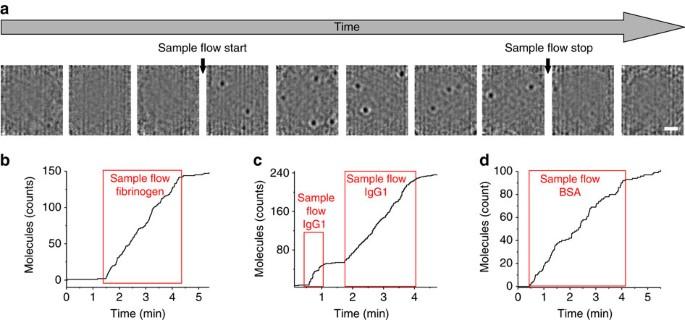Figure 4: Time series of single protein detection. (a) Time series of differential images acquired during the detection of fibrinogen. The first three differential images show the background signal before introducing the analyte. When the sample is pumped into the proximity of the sensor surface, clear and discrete spots of molecular bindings appear in the image. After the sample flow is stopped, the differential images show only the background noise again. Scale bar is the same for all frames and corresponds to 1 μm. (b) Temporal kinetics of fibrinogen detection (corresponding toSupplementary Movie 1). (c) Temporal kinetics of IgG1 detection (corresponding toSupplementary Movie 2). (d) Temporal kinetics of BSA detection (corresponding toSupplementary Movie 3). Figure 4: Time series of single protein detection. ( a ) Time series of differential images acquired during the detection of fibrinogen. The first three differential images show the background signal before introducing the analyte. When the sample is pumped into the proximity of the sensor surface, clear and discrete spots of molecular bindings appear in the image. After the sample flow is stopped, the differential images show only the background noise again. Scale bar is the same for all frames and corresponds to 1 μm. ( b ) Temporal kinetics of fibrinogen detection (corresponding to Supplementary Movie 1 ). ( c ) Temporal kinetics of IgG1 detection (corresponding to Supplementary Movie 2 ). ( d ) Temporal kinetics of BSA detection (corresponding to Supplementary Movie 3 ). Full size image Figure 3i plots the relationship between the measured iSCAT contrast and the molecular weights of the four proteins. Here, we expect a linear relationship if we assume similar indices of refraction and densities for different proteins because the iSCAT signal is proportional to the protein polarizability and therefore its volume. Experimental confirmation of this prediction in Fig. 3i provides further evidence for the robustness of our measurements and interpretation and shows the ability of iSCAT to count a range of clinically relevant proteins. One example of cancer-related biomarkers is CEA, included in this study. Many other biomarkers with typical molecular weight of hundreds of kDa (for example, thyroglobulin, cancer antigen 125) or tens of kDa (for example, prostate-specific antigen, alpha-fetoprotein, vascular endothelial growth factor receptor) [25] are, thus, also readily accessible to iSCAT biosensing. Furthermore, these data indicate that iSCAT can be used to determine the mass of the detected biomolecule within the measurement error although the signal under a given illumination polarization is also sensitive to the particle shape. We anticipate that the slightly increased contrast of IgG1 in Fig. 3i might be due to its asymmetric shape. Performance at different concentrations To verify the practical biosensing capabilities of iSCAT and its applicability to complex surface chemistry, we functionalized a coverslip with a conventional low-fouling poly(ethyleneglycol) surface and anti-IgG1 antibodies and used it to detect different concentrations of IgG1. For a control experiment, IgG1 was labelled with Alexa 647 dye and detected with single-molecule sensitivity via total internal reflection fluorescence (TIRF) microscopy. Here, we carried out the fluorescence detection on the same sensor surface while the iSCAT illumination was temporarily switched off to avoid strong photobleaching. Series of 1, 10 and 100 ng ml −1 concentrations of IgG1+Alexa647 in phosphate-buffered saline (PBS) were pumped for 1 min at 500 nl min −1 to the close proximity of the detection area through the opening of a pulled glass micropipette (see Methods). TIRF and iSCAT images were recorded subsequently. The red and black curves in Fig. 5a–c display time series of individual binding events for iSCAT and TIRF, respectively. In all cases, we find a stable baseline prior to the detection followed by a rapid increase in the binding rate, ranging from 5 to 150 bindings per minute for different concentrations. 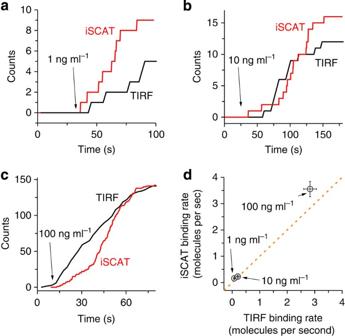Figure 5: IgG binding at different concentrations. Kinetics of iSCAT and fluorescence signals (measured consecutively) for IgG1 solutions with concentrations (a) 1 ng ml−1, (b) 10 ng ml−1and (c) 100 ng ml−1. (d) Plot of the iSCAT binding rate versus the binding rate determined by TIRF. The diagonal line marks a slope of 1. Error bars indicate the statistical error resulting from the total number of detected molecules. Figure 5d shows a linear relation between the binding rates measured by iSCAT and TIRF. Considering the single-molecule sensitivity of TIRF detection, this outcome provides another strong independent evidence that our label-free iSCAT biosensor has reached the single-molecule detection level. Moreover, the data show that an amount of analyte as small as 3 amol, corresponding to a concentration of 6 pM (1 ng ml −1 ), was sufficient for achieving a good SNR. The upper limit of detection in the low nanomolar range is common to all single-molecular approaches and can be easily extended by using dilution series or a complementary less-sensitive method. Figure 5: IgG binding at different concentrations. Kinetics of iSCAT and fluorescence signals (measured consecutively) for IgG1 solutions with concentrations ( a ) 1 ng ml −1 , ( b ) 10 ng ml −1 and ( c ) 100 ng ml −1 . ( d ) Plot of the iSCAT binding rate versus the binding rate determined by TIRF. The diagonal line marks a slope of 1. Error bars indicate the statistical error resulting from the total number of detected molecules. Full size image Specific vs nonspecific response We have demonstrated the exquisite sensitivity of iSCAT for detecting single small proteins and its ability to deliver conventional biosensing kinetics curves. A working sensor, however, is required to detect a particular analyte molecule in a heterogeneous solution of other entities, which could be present at much higher concentrations than the molecule of interest. The concentration ratio of target to background molecules in biological fluids can be as small as 10 −8 (ref. 26 ). The specificity of biosensors and discrimination against the unwanted signal of background proteins are usually achieved via surface chemistry and the binding selectivity [27] , [28] . In practice, a small fraction of the background proteins do bind to the surface, creating a residual signal. Existing biosensor devices account for this background by first measuring it without the sample of interest and then subtracting a reference signal [29] . To demonstrate the potential application of this approach for iSCAT sensing, we performed a proof-of-principle experiment, where CEA was detected in the presence of a high concentration of IgG1. Here, the surface was functionalized with monoclonal antibodies that bind specifically to CEA (see Methods). In Fig. 6a we display the histogram of Fig. 3b for CEA in pure buffer. In Fig. 6b , we plot the histogram (black) from the detection of 20 ng ml −1 of CEA in a mixture with 50 μg ml −1 of IgG. The observation that the histograms of the specific and nonspecific species begin to overlap implies that the dynamic range of our specificity corresponds to 2 × 10 3 in this case. As a further check, in Fig. 6d we present the data from a measurement with five times lower concentration of IgG1 (10 μg ml −1 ). We find that here the CEA signal clearly stands out. 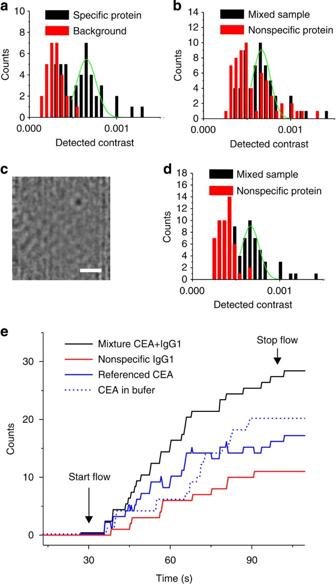Figure 6: Specific detection in a mixed sample. (a) Histogram of iSCAT signal from CEA (black) versus background of pure buffer (red). This is the same figure asFig. 3c. (b) Corresponding histogram of the contrasts measured in a sample with abundant nonspecific proteins (red), and in a mixture of CEA and nonspecific protein (black). (c) Example of a differential iSCAT image after introducing CEA in a mixture with abundant nonspecific proteins. Scale bar, 1 μm. (d) Same as (b) but with five times lower concentration of nonspecific proteins. (e) Kinetics of specific detection in a mixed sample (black), nonspecific abundant IgG1 proteins (red) and the difference between the black and red traces (blue). The dotted blue trace plots the kinetics of CEA in pure buffer for comparison. Figure 6: Specific detection in a mixed sample. ( a ) Histogram of iSCAT signal from CEA (black) versus background of pure buffer (red). This is the same figure as Fig. 3c . ( b ) Corresponding histogram of the contrasts measured in a sample with abundant nonspecific proteins (red), and in a mixture of CEA and nonspecific protein (black). ( c ) Example of a differential iSCAT image after introducing CEA in a mixture with abundant nonspecific proteins. Scale bar, 1 μm. ( d ) Same as ( b ) but with five times lower concentration of nonspecific proteins. ( e ) Kinetics of specific detection in a mixed sample (black), nonspecific abundant IgG1 proteins (red) and the difference between the black and red traces (blue). The dotted blue trace plots the kinetics of CEA in pure buffer for comparison. Full size image In Fig. 6c we also present an iSCAT biosensor image of the mixture corresponding to the measurement of Fig. 6b . The image verifies that the background stays quiet despite the diffusion of thousands of IgG1 molecules through the volume defined by the field of view and the depth of focus of our microscope objective. To understand this situation, it is important to note that the interferometric nature of iSCAT leads to alternating contrasts as a function of displacement along the optical axis [20] so that the signal from proteins moving in this direction averages out. Furthermore, diffusing molecules do not reside at the sensor surface long enough to be registered. The black trace in Fig. 6e displays the kinetics of the biosensor signal in a mixture, whereas the blue trace presents the same data after subtracting the residual IgG1 background given by the red trace. The facts that the blue trace stands out well above the nonspecific background (red) and that it agrees with the kinetics of CEA in buffer (dotted blue trace) confirm that the referencing strategy works. We point out that the residual nonspecificity is not an artefact of iSCAT, but it is associated with the performance and purity of the CEA monoclonal antibody used in this demonstration. Indeed, as for other common biosensors [8] , [9] , [10] , [11] , [12] , [13] , [14] , [15] , [16] , the specificity of an iSCAT sensor relies on the choice of surface chemistry [26] . To this end, the value of 2 × 10 3 demonstrated here is not a fundamental limit for iSCAT sensing. Other combinations of analyte and antibody or future developments in surface chemistry could yield better performance. Furthermore, the intrinsic limit of the obtained specificity is determined by the noise on the signal and background histograms (see, for example, Fig. 6b ). Considering that this is dictated by the shot noise of the total number of recorded molecules, it can be increased by longer detection times. It is also worth mentioning that current state-of-the-art high-end bioanalysis could take up to several hours [30] . In the case of less-sensitive methods such as surface plasmon resonance sensors, the better statistics is offered by the large concentrations involved. Super-resolution imaging of protein-binding sites In addition to the ultimate biosensor performance of detecting individual analyte molecules, our recordings register the spatial coordinates of each molecule with nanometer precision. The symbols in Fig. 7a represent the iSCAT image of a single fibrinogen while the surface plot depicts a two-dimensional Gaussian fit. The SNR of the order of 10 allows localization of the centre of the Gaussian peak with a precision of 5 nm, which agrees with the theoretical limit of localization within 10% (ref. 31 ). Since in our experiment the proteins land one by one, we can extend this procedure to acquire super-resolution iSCAT images of the binding process, whereby subsequent arrival times are used to identify the signals of individual molecules [32] . 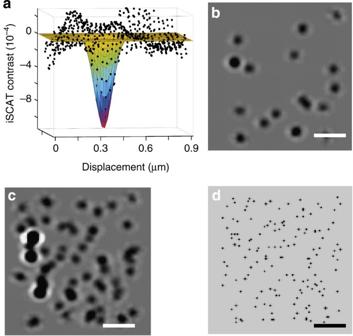Figure 7: Super-resolution imaging. (a) An iSCAT image of a molecule fitted with a two-dimensional Gaussian, yielding a localization precision of 5 nm. (b) Images of individual molecules accumulated in 15 s. (c) Images of individual proteins accumulated in 60 s. (d) Super-resolution image, showing the localized positions of the binding events accumulated in 150 s. Scale bar, 1 μm. Figure 7b,c shows iSCAT images accumulated after 15 and 60 s of detection, and Fig. 7d displays the localization map of all molecules accumulated in 150 s. Each position of the localization map therefore corresponds to one binding site available on the surface. This provides the first generalization of the recent super-resolution microscopy methods [33] , [34] to the study of nonfluorescent samples such as novel biointerfaces and their function [35] . Figure 7: Super-resolution imaging. ( a ) An iSCAT image of a molecule fitted with a two-dimensional Gaussian, yielding a localization precision of 5 nm. ( b ) Images of individual molecules accumulated in 15 s. ( c ) Images of individual proteins accumulated in 60 s. ( d ) Super-resolution image, showing the localized positions of the binding events accumulated in 150 s. Scale bar, 1 μm. Full size image We have shown that careful consideration of the quantities involved and proper experimental procedure makes it possible to detect the Rayleigh scattering of a single unlabelled biomolecule in a straightforward and direct optical measurement. This approach can count proteins, is compatible with a wide range of functionalization methods, provides nanoscopic spatial information of binding events, can be easily parallelized, and is not limited to confined optical fields. In addition, iSCAT sensing can be used to visualize the motion of proteins (ref. 36 ) and monitor the association and dissociation kinetics of biomolecules and study their cooperative interactions [37] because it does not suffer from photobleaching. The sensitivity of iSCAT in our experiment was determined by the pixel well depth of the camera. Considering that the fundamental limit of this method is set by photon shot noise, it can be improved at higher incident powers or integration times. This would allow one to detect yet smaller biomolecules such as microRNA [38] or environmental pollutants. Higher signal-to-noise ratios might also open the door to extracting the absolute molecular mass, shape and orientation of single molecules via the measurement of their polarizabilities. These features and its ease of instrumentation may allow iSCAT biosensing to contribute to early clinical diagnostics of small proteins that have been identified as biomarkers of various diseases such as cancer [25] . Materials Poly-ethyleneglycol-coated coverslips with NHS coupling chemistry for covalent immobilization of proteins were purchased from MicroSurfaces, Inc., TX, USA. Fibrinogen from human plasma, mouse-IgG1 (whole antibody), goat-anti-mouse-IgG1 (whole antibody), mouse-IgG1 labelled with Alexa Fluor 647 and ultrapure BSA were purchased from Life Technologies GmbH, Germany. CEA from human fluids and monoclonal anti-CEA were obtained from Sigma-Aldrich. PBS, sodium acetate buffer (pH 5.2) and other common chemicals were obtained from Sigma-Aldrich. Experimental set-up The output of a continuous-wave diode laser (wavelength 405, Toptica, Inc.) was intensity stabilized to better than 3 × 10 −4 using a proportional-integral-derivative control loop. The incident beam was circularly polarized, directed through a 70:30 beam splitter, and focused at the back focal plane of a microscope objective (NA=1.46, Zeiss). Functionalized surface of a glass coverslip was placed in the focus of the microscope objective and the focal position was stabilized with an active feedback loop. The full-width at half-maximum of the microscope point spread function was typically between 190 and 200 nm. A narrow field of view of 4.5 μm × 4.5 μm was illuminated with a power of 10 mW. The light reflected and scattered at the glass/water interface was collected with the same microscope objective and imaged via the 70:30 beam splitter on a fast CMOS camera (Photonfocus, AG). An area of 128 × 128 pixels of the camera was acquired at the frame rate of 3,000 frames per second. Experimental procedure A pure diluting buffer was placed in a plexiglass cuvette of 5 ml volume on the coverslip. Micropipettes were pulled from a thin-wall glass capillary (OD 1 mm/ID 0.75 mm) to obtain flat ends with an opening diameter of 5 μm. The micropipette was positioned at ~10 μm above the coverslip surface and in close proximity to the iSCAT field of view. This position was chosen to avoid visible artefacts or fringes in the image. The characteristic volume between the pipette tip and the surface was in the picoliter range. This volume results in a diffusion time of ~200 ms for the analyte molecules to reach the sensor surface. The minimum flow rate required to maintain constant concentration in the vicinity of the sensor surface was of the order of nl min −1 . Higher flow rates of 500 nl min −1 driven by a conventional syringe pump were used to maintain a stable pulse-free flow. Coverslips were coated with poly(ethyleneglycol) brush (thickness of 2-3 nm) with NHS reactive groups (10 7 binding sites within the field of view). Coated coverslips were either used directly to capture BSA, IgG1 or fibrinogen or further functionalized with a high concentration of anti-IgG1 or anti-CEA. In the first case, the cuvette was filled with a buffer of sodium acetate. A concentration of 200 ng ml −1 of the protein solution in SA buffer was loaded in the micropipette. After acquiring 100 frames of the baseline signal the sample was pumped for a few minutes in order to clearly observe the difference of the surface scattering before and during the detection. Once the pumping was stopped, the analyte molecules diffused and diluted in the cuvette on the time scale of seconds, decreasing the concentration at the surface by typically 3 orders of magnitude (depending on the duration of pumping). In the case of specific IgG1 detection, the sensor surface was incubated with 20 μg ml −1 solution of anti-IgG1 in SA buffer for 20 min, followed by 20 min incubation in NHS deactivating buffer. The functionalized coverslip was then mounted on the set-up, the cuvette was filled with PBS buffer and the micropipette with the corresponding target concentration (1, 10 or 100 ng ml −1 ) of IgG1 dissolved in PBS was placed into the cuvette. In the case of specific CEA detection, the sensor surface was incubated with 10 μg ml −1 solution of anti-CEA in SA buffer for 20 min followed by 20 min incubation in NHS deactivating buffer. The functionalized coverslip was then mounted on the set-up, the cuvette was filled with PBS buffer and the micropipette with 20 ng ml −1 concentration of CEA dissolved in PBS was placed into the cuvette. For the specificity experiment two micropipettes were used, one containing 10 or 50 μg ml −1 solution of IgG1 in PBS, and the other containing a mixed sample of 50 μg ml −1 of IgG and 20 ng ml −1 of CEA for comparison. Noise and visibility analysis Noise and visibility can be derived from the quantitative estimate of our experimental parameters. We illuminate 20 μm 2 of the sensor surface with 10 mW incident power, which amounts to 15 μW per area of DLS. Considering the photon energy at a wavelength 405 nm of 5 × 10 −19 J, P inc =3 × 10 13 photons s −1 DLS −1 . For a scattering cross-section of σ =10 11 μm 2 , collection efficiency of 35%, losses of 75% in the detection path (that is, 25% throughput) and area of DLS= π (100 nm) 2 in our experimental set-up, the detector receives . Assuming r 2 =0.006 for the reflectivity of the glass–water interface, the powers in the reference beam and the interferometric term become P ref =6 × 10 −3 × 0.25 P inc =1.5 × 10 −3 P inc =4.5 × 10 10 photons s −1 DLS −1 and , respectively. Our experimental set-up is configured to provide × 300 magnification with a camera pixel size of 10 μm. Therefore, the area of a DLS on the camera corresponds to . Considering a quantum efficiency QE=0.25 for the CMOS camera at a wavelength of 405 nm and exposure time of t =0.2 ms, the reference and interferometric signals received by each pixel are . The well depth of the CMOS camera was , limiting the maximum incident power in our experiment. In a similar fashion, we can calculate the contribution of the iSCAT signal as To achieve a better shot-noise limit, we averaged many frames. For the detection of the smallest protein (BSA) the signal yields 11,200 P int per pixel=2 × 10 5 photoelectrons, while the standard deviation of the signal fluctuation becomes In this case, we obtain , which is in good agreement with our experimental results. Data analysis In order to visualize changes in the scattering signal and their spatial distribution, we continuously processed sets of several hundreds of consecutive frames and extracted the image of the surface roughness (see Fig. 2a–d ). Differential images were then calculated from two sets of images separated by a temporal delay of 300 ms and a running average was used to accomplish continuous acquisition of differential images. All differential images were processed with a routine that searched for local minima over a region of the size of a DLS on the camera. Any mechanical drifts and instabilities were negligible on the time scale of up to 5 s. How to cite this article: Piliarik, M. et al. Direct optical sensing of single unlabelled proteins and super-resolution imaging of their binding sites. Nat. Commun. 5:4495 doi: 10.1038/ncomms5495 (2014).